Prosody cues word order in 7-month-old bilingual infants A central problem in language acquisition is how children effortlessly acquire the grammar of their native language even though speech provides no direct information about underlying structure. This learning problem is even more challenging for dual language learners, yet bilingual infants master their mother tongues as efficiently as monolinguals do. Here we ask how bilingual infants succeed, investigating the particularly challenging task of learning two languages with conflicting word orders (English: eat an apple versus Japanese: ringo-wo taberu ‘apple.acc eat’). We show that 7-month-old bilinguals use the characteristic prosodic cues (pitch and duration) associated with different word orders to solve this problem. Thus, the complexity of bilingual acquisition is countered by bilinguals’ ability to exploit relevant cues. Moreover, the finding that perceptually available cues like prosody can bootstrap grammatical structure adds to our understanding of how and why infants acquire grammar so early and effortlessly. When hearing speech in an unfamiliar language, the listener has no explicit information signalling the underlying structural rules that speakers use to produce sentences. Similarly, acquiring the grammatical properties of the native language constitutes a seemingly formidable learning problem for young infants [1] , [2] , [3] , and the means by which infants succeed are only beginning to be understood. Acquiring grammar in a bilingual environment where the two languages have conflicting word orders like English and Japanese is an even more challenging task, and the mechanisms that bilingual infants use to solve this problem are not yet known [4] . As the majority of the world’s population today is exposed to multiple languages from birth [4] , a better understanding of their early cognitive development might have considerable impact on social and educational policies worldwide. Even a rudimentary knowledge of word order is of particular relevance for language development, because its successful mastery might have a cascading effect on learning even before infants can actively use this knowledge in production. Knowing the canonical word order might allow infants to parse utterances into constituents and assign grammatical functions to unfamiliar words, making it easier to identify their referents and learn their meanings. The languages of the world differ in their basic word order type in systematic ways. The basic word order of a language is defined by the relative order of the verb (V) and its object (O). This order, in turn, correlates with the relative order of other constituents [5] . In VO languages, like English, Italian or Spanish, for example, prepositions and articles typically precede nouns ( to London , the house ), whereas in OV languages, like Japanese, Turkish or Basque, they most often follow them (Japanese: Tōkyō ni ‘Tokyo to’; Basque: etxe bat ‘house one/a’). Thus, in VO languages, functors, that is, grammatical morphemes such as prepositions, articles, pronouns and so on (for example, to, in, it, the and so on), typically occur in phrase-initial positions, while in OV languages, they usually occupy phrase-final positions. Monolingual infants can use functors as anchors to segment speech into syntactically relevant chunks, from which the basic word order of a language might be deduced [6] , [7] . Functors provide a reliable, systematic and easily recognizable signal, because they are more frequent than content words [6] , [8] and they have distinct perceptual characteristics [9] , [10] , [11] , [12] , [13] . Further, the relative order of function words and content words strongly correlates with basic word order [5] . Consequently, tracking the positions of the most frequent words in the input can help infants acquire more general knowledge about word order. Indeed, after several months of experience with their native language, Italian infants parse a continuous artificial speech stream with alternating frequent and infrequent words into chunks starting with a frequent word, followed by an infrequent word, mirroring the function word-initial word order of Italian ( a Roma ‘to/in Rome’), whereas Japanese infants prefer the opposite, function word-final order, characteristic of Japanese ( Tōkyō ni ‘Tokyo to’) [6] . However, for bilingual infants growing up with a VO and an OV language at the same time, frequency alone is not sufficient, as both frequent word-initial and frequent word-final phrases occur in their input (from the VO and the OV language, respectively). Phrase-level prosody provides an additional cue, which might be informative, as it correlates with word order and is readily available in the acoustic signal [14] . Specifically, in VO languages, prosodic prominence is realized as a durational contrast, with the semantically and syntactically prominent content word being lengthened as compared with the functor, resulting in an iamb or weak–strong pattern ( to Ro me ). In OV languages, prosodic prominence is implemented as a pitch/intensity contrast, with the prominent content word being higher in pitch and/or intensity than the functor, giving rise to a trochee or strong–weak pattern (‘ To kyo ni ). A sensitivity in bilingual infants to prosodic prominence could be used, together with word frequency, to disambiguate word order in the two native languages [14] . Results from our studies on bilingual infants indicate that they are indeed able to exploit these two cues to select the word order characterizing each of their languages. Characterizing bilinguals infants We tested whether bilingual infants growing up with a VO language (English) and an OV language (one of Japanese, Korean, Hindi/Punjabi, Farsi or Turkish) exploit prosodic cues in conjunction with word frequency to discriminate the typical orders of the two languages. As the prosodic and frequency patterns have not previously been empirically verified for all of the OV languages that we used, we first established that those properties do exist in the previously undescribed languages (see Figs 1 and 2 , as well as the Methods). Twenty-four infants were tested in an artificial grammar learning task. Familiarization consisted of a 4-min-long speech stream with alternating frequent and infrequent words concatenated without pauses (structure: … A X B Y A X B Y A X B Y…, stream: … fi ra ge ro fi du ge ka fi to ge ri…; Fig. 3 ; for further details see also ref. 6 ). Frequent words (for example, ‘fi’) were nine times more frequent than infrequent ones (for example, ‘ra’). The onset and the end of the stream were ramped in amplitude to mask phase information, rendering the stream ambiguous between a frequent word-initial, that is, (frequent–infrequent) (FI) and a frequent word-final, that is, (infrequent–frequent) (IF) parse ( Fig. 3 ). We synthesized the familiarization stream with OV prosody for one group of infants ( n =12), using high pitch (224 Hz) on the prominent infrequent words and low pitch (200 Hz) on the non-prominent frequent words (see the Supplementary Methods and Supplementary Audio 1-4 ). For another group of infants ( n =12), we used VO prosody, where the prominent infrequent words were long (144 ms), the non-prominent frequent words were short (120 ms; see Supplementary Methods and Supplementary Audio 1-4 ). Pitch and duration values were based on actual measurements in real speech samples [14] (see also Fig. 2 and the Methods). After familiarization, both groups of infants were tested on eight test items constructed using the same underlying structure as that of the familiarization stream ( Fig. 3 ). Four had FI order (for example, fi fo ge bi ), the other four IF order (for example, ka fi pa ge ). They all had flat prosody and equal syllable durations (see Supplementary Methods and Supplementary Audio 1-4 ). We used the head turn preference procedure to measure infants’ looking times to the test items ( Fig. 4 ). 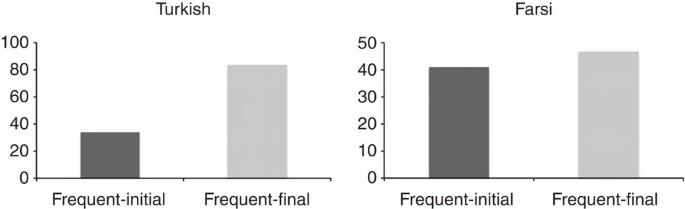Figure 1: The number of frequent word-initial and frequent word-final phrases at utterance edges in child-directed corpora of Farsi and Turkish. Dark grey bars indicate the number of frequent word-initial phrases; light grey bars indicate the number of frequent word-final phrases. Theyaxes indicate the percentage of multiword utterances, where the maximum is 200%, as each utterance contributes two data points (its beginning and its end). Figure 1: The number of frequent word-initial and frequent word-final phrases at utterance edges in child-directed corpora of Farsi and Turkish. Dark grey bars indicate the number of frequent word-initial phrases; light grey bars indicate the number of frequent word-final phrases. The y axes indicate the percentage of multiword utterances, where the maximum is 200%, as each utterance contributes two data points (its beginning and its end). 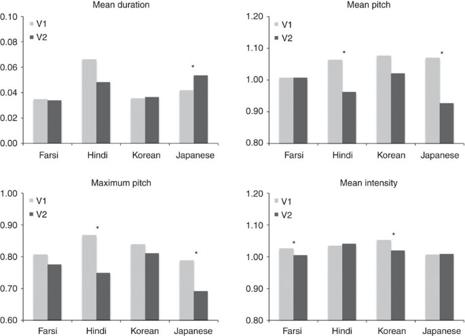Figure 2: Acoustic measures. The mean duration, mean pitch, maximum pitch and mean intensity of the stressed vowels of content words (V1; light grey) and functors (V2; dark grey) within phonological phrases in Farsi, Hindi, Japanese and Korean are shown. Theyaxes represent values normalized to the carrier sentences in which the phrases occurred. Asterisks indicate statistically significant differences (two-tailed, paired samplet-tests, significance set toP=0.0125 per language to correct for multiple comparisons: mean duration for Japaneset(30)=4.62,P=0.0001; mean pitch for Hindit(48)=3.71,P=0.0005 and Japaneset(30)=2.98;P=0.0057; maximum pitch for Hindit(48)=6.37,P<0.0001 and Japaneset(30)=2.80,P=0.0088; mean intensity for Farsit(31)=4.57,P=0.0001 and Koreant(19)=4.15,P=0.0005) between V1 and V2. In addition, a two-tailed, paired samplet-test pooling together data from all four languages was also performed and yielded the following results: no statistically significant difference between V1 and V2 for duration (V1: 0.048, V2: 0.044;t(131)=1.291, NS), marginally significantly higher intensity for V1 than for V2 (V1: 1.029, V2: 1.021;t(131)=1.922,P=0.056), higher mean pitch for V1 than for V2 (V1: 1.053, V2: 0.973;t(131)=4.027,P<0.0001), and higher maximum pitch for V1 than for V2 (V1: 0.831, V2: 0.751;t(131)=5.870,P<0.0001). In sum, the OV languages utilize higher pitch and, sometimes, higher intensity on the initial element to mark prosodic prominence. Full size image Figure 2: Acoustic measures. The mean duration, mean pitch, maximum pitch and mean intensity of the stressed vowels of content words (V1; light grey) and functors (V2; dark grey) within phonological phrases in Farsi, Hindi, Japanese and Korean are shown. The y axes represent values normalized to the carrier sentences in which the phrases occurred. Asterisks indicate statistically significant differences (two-tailed, paired sample t -tests, significance set to P =0.0125 per language to correct for multiple comparisons: mean duration for Japanese t (30)=4.62, P =0.0001; mean pitch for Hindi t (48)=3.71, P =0.0005 and Japanese t (30)=2.98; P =0.0057; maximum pitch for Hindi t( 48)=6.37, P <0.0001 and Japanese t (30)=2.80, P =0.0088; mean intensity for Farsi t (31)=4.57, P =0.0001 and Korean t (19)=4.15, P =0.0005) between V1 and V2. In addition, a two-tailed, paired sample t -test pooling together data from all four languages was also performed and yielded the following results: no statistically significant difference between V1 and V2 for duration (V1: 0.048, V2: 0.044; t (131)=1.291, NS), marginally significantly higher intensity for V1 than for V2 (V1: 1.029, V2: 1.021; t (131)=1.922, P =0.056), higher mean pitch for V1 than for V2 (V1: 1.053, V2: 0.973; t (131)=4.027, P <0.0001), and higher maximum pitch for V1 than for V2 (V1: 0.831, V2: 0.751; t (131)=5.870, P <0.0001). In sum, the OV languages utilize higher pitch and, sometimes, higher intensity on the initial element to mark prosodic prominence. 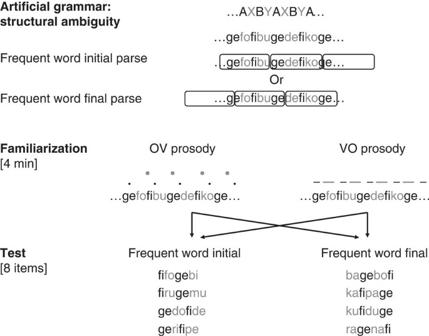Figure 3: The material used in Experiments 1 and 2. Frequent (dark grey) and infrequent (light grey) words strictly alternate in the artificial grammar, giving rise to two possible parses. In one, the basic unit starts with a frequent word and ends in an infrequent word (FI), whereas in the other, the basic unit starts with an infrequent word and ends in a frequent word (IF). To create the familiarization stream, prosody characteristic of OV languages, that is, a high-low pitch contrast, was added to the alternating structure for one group of infants in Experiment 1 and for all infants in Experiment 2, while VO prosody, that is, a short-long durational contrast, was used for a second group of infants in Experiment 1. Test items were identical for all groups. Half had an FI structure, the other half an IF structure, with no prosody added. Full size image Figure 3: The material used in Experiments 1 and 2. Frequent (dark grey) and infrequent (light grey) words strictly alternate in the artificial grammar, giving rise to two possible parses. In one, the basic unit starts with a frequent word and ends in an infrequent word (FI), whereas in the other, the basic unit starts with an infrequent word and ends in a frequent word (IF). To create the familiarization stream, prosody characteristic of OV languages, that is, a high-low pitch contrast, was added to the alternating structure for one group of infants in Experiment 1 and for all infants in Experiment 2, while VO prosody, that is, a short-long durational contrast, was used for a second group of infants in Experiment 1. Test items were identical for all groups. Half had an FI structure, the other half an IF structure, with no prosody added. 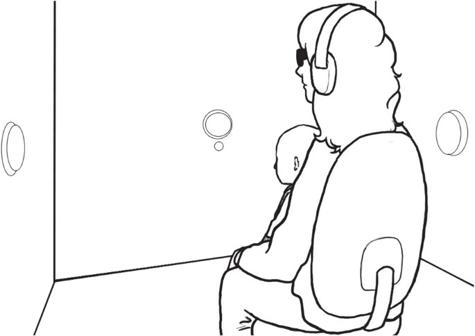Figure 4: The head turn preference paradigm. Infants are seated on a parent’s lap in a sound-attenuated room with a central fixation light in front of them and two fixation lights on the side. During familiarization, the speech stream is played symmetrically from both sides of the room and the lights blink contingently on the infant’s looking behaviour, but independently of the sound. During test, each item is presented from either the left or the right side of the room, counterbalanced across the eight test items. The light on the corresponding side blinks contingently on the infant’s looking. The session is videotaped and coded off-line to measure the time infants spend looking at and listening to the test items in the two experimental conditions. Full size image Figure 4: The head turn preference paradigm. Infants are seated on a parent’s lap in a sound-attenuated room with a central fixation light in front of them and two fixation lights on the side. During familiarization, the speech stream is played symmetrically from both sides of the room and the lights blink contingently on the infant’s looking behaviour, but independently of the sound. During test, each item is presented from either the left or the right side of the room, counterbalanced across the eight test items. The light on the corresponding side blinks contingently on the infant’s looking. The session is videotaped and coded off-line to measure the time infants spend looking at and listening to the test items in the two experimental conditions. Full size image Infants familiarized with OV prosody showed longer looking times for the IF test items than for the FI ones, whereas infants familiarized with VO prosody showed the opposite pattern ( Fig. 5 ). An analysis of variance with Prosody (OV/VO) as a between-subject and test items (FI/IF) as a within-subject factor showed a significant interaction ( F (1,22)=11.000, P =0.003; pair-wise Scheffé post hoc tests for the FI/IF comparisons: P =0.025 for OV prosody and P =0.031 for VO prosody). Bilingual infants can thus use prosody to identify the relevant word order in each of their two native languages. 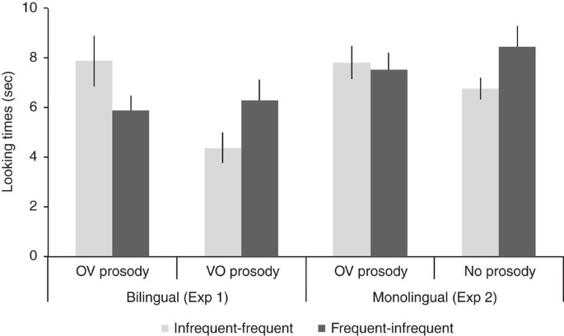Figure 5: Looking time results for Experiment 1 and 2. Thexaxis shows the experimental groups. Theyaxis represents infants’ looking times in seconds. The light grey bars indicate looking times to the IF test items, the dark grey bars to the FI items. The error bars represent the s.e. of the mean. Figure 5: Looking time results for Experiment 1 and 2. The x axis shows the experimental groups. The y axis represents infants’ looking times in seconds. The light grey bars indicate looking times to the IF test items, the dark grey bars to the FI items. The error bars represent the s.e. of the mean. Full size image Characterizing monolingual infants Is the sensitivity to the prosodic patterns a result of bilingual exposure or is it a more general perceptual grouping mechanism, guiding infants’ word order preferences even without prior experience? On the one hand, there is evidence suggesting that the auditory system automatically groups elements contrasting in pitch/intensity as prominence-initial (that is, trochaic) and elements contrasting in duration as prominence-final (that is, iambic), independently of language experience [15] . The trochaic grouping on the basis of pitch information appears to be particularly salient, as even rats have been demonstrated to show this, but not the iambic bias [16] . It is, therefore, possible that, at least at the beginning of development, before the native language is fully mastered, the specific prosodic pattern heard guides the choice of word order, even if it is absent from or unlike that of the native language. On the other hand, recent results indicate that language experience may influence prosodic grouping [17] , [18] . Our bilingual results are compatible with both hypotheses. Therefore, in Experiment 2, we tested 7-month-old monolingual English-exposed infants using the OV prosody condition of Experiment 1, that is, a prosody unfamiliar to the infants, as well as in a no prosody control (the same artificial grammar with no pitch or durational cues, that is, constant pitch of 200 Hz and constant duration of 120 ms, as in ref. 6 ). The familiar VO prosody condition was not tested. Recent work with monolingual French infants [19] , a language with word order and phrasal prosody similar to English [14] , has already revealed that monolingual infants can use trochaic prosody to guide word order preferences. Also, a VO condition would not allow us to tease apart the effects of familiarity and a universal iambic-trochaic bias. The results of the unfamiliar OV prosody condition, by contrast, are informative: (i) if an IF order preference is obtained, it can only result from a language-independent prosodic principle, as English provides neither prosodic, nor word frequency cues to this order; (ii) if an FI preference is found, then monolinguals ignore the prosodic cue and use only word frequency; and (iii) the absence of a preference would indicate that monolinguals are sensitive to the conflict of the two cues. The no prosody condition assessed English monolinguals’ baseline preference for the word frequency cue alone, testing whether the results of Gervain et al. [6] with Italian monolinguals can be generalized to their English-exposed peers. In the unfamiliar OV prosody condition, monolingual English infants did not show significantly different looking times to the FI and IF test items (mean: 7.51 and 7.82s, respectively; Fig. 5 ). However, the predicted preference for FI items was observed in the no prosody condition (FI and IF mean: 8.44 and 6.77s, respectively; Fig. 5 ). An analysis of variance with Prosody (OV/none) as a between-subject and test items (FI/IF) as a within-subject factor showed a significant interaction ( F (1,45)=4.3177, P =0.0435; pair-wise Scheffé post hoc tests for the FI/IF comparisons: NS for OV prosody and P =0.0259 for the no prosody condition) This suggests that English monolinguals, like their Italian and Japanese peers, can use word frequency as a unique cue to word order. Further, they are sensitive to the conflict between word frequency (cuing the FI order) and the non-native OV prosody (cuing the IF order). Importantly, the latter is not a sufficiently strong cue for them at this age to induce a preference for the corresponding IF order. In two artificial grammar learning experiments with 7-month-old infants, we have shown that bilinguals exposed to an OV and a VO language simultaneously are able to use relevant prosodic information as a cue to the corresponding order of frequent and infrequent items. That these findings were obtained across a variety of different English-OV language pairs indicates a robust, generalizable phenomenon. These results are crucial to our understanding of bilingual development, because they identify prosodic bootstrapping as a mechanism that bilingual infants use to solve the complex learning problem they encounter. Our findings with monolinguals also suggest that at least by 7 months, basic word order preference as cued by word frequency is well established and cannot (or can no longer) be fully reversed by prosody. The ability to determine the relative order of frequent and infrequent items in the native language(s) on the basis of prosody provides infants with an important stepping stone towards acquiring the relative order of basic constituents such as verbs and objects. Indeed, we have shown that this latter correlates with the relative order of frequent and infrequent words in corpora of the languages tested ( Fig. 1 and ref. 6 ) as well as in other languages [8] , [13] . Prosody is, therefore, a useful cue to the acquisition of basic word order phenomena, as proposed before [14] , [20] . Importantly, our study investigates the first steps into language structure. Word order is a complex linguistic phenomenon, which takes years to master in its full complexity [21] . Further work will be necessary to explore how the beginnings uncovered in our study develop into full-fledged competence. Nonetheless, by showing that bilingual infants use two distinct perceptual cues, we provide some of the strongest evidence to date that the prosodic properties of the linguistic signal have a crucial role in acquiring language structure [13] . How does sensitivity to prosodic patterns arise? Existing studies with monolingual infants mostly tested these infants’ grouping preferences, not the use of this preference as a potential bootstrapping cue. In Yoshida et al. [22] study with monolingual OV and monolingual VO populations (Japanese and English, respectively), language-specific prosodic grouping was not observed at 5–6 months, but it appeared at 7–8 months. These authors did not test pitch/intensity, only duration as a cue, and the stimuli consisted of pure tones, not syllables. Using speech sequences, Bion et al. [18] found prosodic grouping in monolingual Italian infants at 7 months for the pitch/intensity contrast, but not for the durational one. The two studies used stimuli of different nature and complexity, that is, pure tones versus speech, which might explain why a duration-based grouping preference was found in one VO-exposed population (English infants in the Yoshida et al. [22] study), but not in the other (Italian infants in the Bion et al. [18] study). Further, recent evidence with animals suggests that trochaic grouping on the basis of pitch might be an automatic and universal feature of the mammalian auditory system, as rats also exhibit this grouping preference, whereas iambic grouping on the basis of duration might require language experience [16] . This asymmetry might explain why the pitch-based trochaic grouping preference, typical of OV languages, is found in the VO-exposed Italian infant population. Bilingual infants’ sensitivity to prosody has not previously been tested. Our results are the first to show that by 7 months of age, bilingual infants can also exploit prosody as a cue to word order. However, as sensitivity to prosodic grouping has never been tested in infants younger than 4–5 months, it remains an open question whether monolingual and bilingual infants have an initial broad sensitivity to different cues, including prosody, or whether sensitivity to these cues develops as a function of language exposure. One possible way to test these alternatives is to investigate whether monolingual infants exposed to languages that have mixed word orders, such as Dutch or German, remain sensitive to prosody. In Dutch and German, both OV and VO orders are possible in some phrases depending on the syntactic and pragmatic context (for example, Dutch VO: op de trap ‘up the stairs’ versus OV: de trap op ‘the stairs up’). Importantly, the two orders are realized with their characteristic prosodies, that is, a pitch/intensity contrast for OV ( de ‘trap op ) and a durational contrast for VO ( op de trap ) [14] . Monolingual infants exposed to a mixed VO–OV language might also use prosody to discriminate between syntactic and pragmatic contexts requiring one or the other order, a hypothesis that remains to be tested empirically. In sum, further research is needed to chart the entire developmental trajectory of the prosodic grouping principle, especially during the very first months of life. A related theoretical question concerns the origin of the correlation between specific prosodic patterns and word orders. Why is phrase-initial (OV) prominence signalled by pitch and/or intensity, and phrase-final (VO) prominence by duration? This question is of considerable interest for future research, as it will not only help elucidate processes of language acquisition, but will also provide insight into how language evolved. We speculate that perceptual grouping biases might originate in speech production. Given the functional anatomy of the articulators and the respiratory system, speech is produced in units known as breath groups [23] . Breath groups are characterized by higher intensity and higher pitched phonation at the beginning and lengthening at the end. Language might have recruited these articulatory, acoustic and auditory properties of phonation to mark prominence in a grammatically relevant way. To conclude, our findings significantly advance knowledge of language acquisition by addressing, for the first time, how bilinguals construct two distinct grammars. By showing that bilingual infants are able to use the prosodic cues to word order, we reveal how the human language learning system flexibly adapts to the linguistic environment it encounters. This discovery helps dismiss the widespread, but unsupported concern that bilingual acquisition leads to language delay. Indeed, it provides evidence of a sensitivity that may lay the foundation for some of the cognitive advantages previously reported among bilinguals [24] , [25] . Further, it demonstrates how studying bilingual infants can reveal mechanisms of language acquisition, and ultimately language evolution, not readily apparent in studies of only a monolingual population. Corpus analysis One assumption underlying our hypothesis is that the sentential position of frequent functors provides a reliable cue to word order in the various OV languages our bilingual participants were exposed to. To test this assumption, we examined infant-directed corpora in Farsi and Turkish, as such measurements already exist in Japanese [6] , and infant-directed corpora are not available for Korean or Hindi/Punjabi. The corpora were taken from the CHILDES database [26] for Farsi [27] and Turkish [28] . For both languages, we extracted the infant-directed adult utterances from the corpora. As one-word utterances are not informative about word order, we discarded these, and used only multiword utterances for our analysis. With this manipulation, we obtained corpora of 10,495 utterances in Turkish and 7,180 utterances in Farsi. We tracked the relative position of frequent and infrequent morphemes at utterance edges, following Gervain et al. ’s [6] method. Utterance boundaries were chosen, as they are perceptually identifiable even by young infants [29] . Frequent and infrequent words (FW and IW, respectively) were defined as having a relative frequency of occurrence higher and lower, respectively, than four predefined thresholds: T 1 =0.01, T 2 =0.005, T 3 =0.0025 and T 4 =0.001. We then identified the first and the last two words of all utterances, that is, two-word ‘phrases’ at the left and right utterance boundaries. If the ‘phrase’ had a (FW IW) order, it was counted as ‘frequent-initial’. If it had an (IW FW) structure, it was counted as ‘frequent-final’. We ignored ‘phrases’ where both words were of the same category, that is, (FW FW) or (IW IW), as they were not informative about the relative order of frequent and infrequent words. The four thresholds yielded similar results, thus we only report results for T 1 ( Fig. 1 ). Acoustic measures Similarly to frequency, we analysed the prosodic patterns of the OV languages the infants were exposed to. Such measurements have previously been reported for Turkish [14] . To ensure that prosody patterned as expected in the remaining OV languages, we conducted acoustic analyses in Hindi, Japanese, Korean and Farsi. We used the same method as Nespor et al. [14] in their study of French, Turkish and German. To summarize briefly, target phrases with a noun followed by a postposition or another functor were constructed in each of the languages (for example, Hindi: sarke neechay head.poss under ‘under the head’). At least four bisyllabic or trisyllabic nouns and two bisyllabic functors were chosen for each language. These were combined to create the target phrases. The phrases were then embedded in an invariant carrier sentence (for example, Hindi: Hindi mein sarke neechay kehte hain. ‘In Hindi under the head is said.’; see the Supplementary Methods for the full list of sentences). Two young female native speakers of each language were recorded producing each sentence twice. As the infants tested in the experiments were recruited from the Vancouver area, we also selected the female native speakers from the communities using each of these languages in Vancouver in order to ensure that the material we analysed was obtained from the same dialect as that of the infants. Speakers were instructed to pronounce the sentences as simple, natural declarative utterances forming one intonational phrase, that is, without pauses. A coder naïve to the purposes of the study measured the duration, mean pitch, pitch maximum and mean intensity of each sentence as well as of the stressed vowel of the noun and the functor. The measures for the vowels were normalized to the respective measures of their carrier sentences to correct for variation in speech rate, fundamental frequency and so on across speakers and languages. The normalized data were entered into t -tests (corrected for multiple comparison) to compare the relative acoustic properties (of the stressed vowels) of the noun and the functor ( Fig. 2 ). Participants Twenty-four (8 females) 7-month-old (mean age: 7.5 months, range: 6.5–9 months) bilingual infants participated in Experiment 1. They received at least 25% exposure to each language (mean: 51% English, 49% OV language) according to the Language Exposure Questionnaire [30] . The number of infants exposed to each specific OV language is as follows: 12 Hindi/Punjabi, 7 Japanese, 3 Korean, 1 Turkish, 1 Farsi. Another 47 7-month-old (mean age: 7.1 months, range: 6.5–8 months) monolingual infants (17 females) participated in Experiment 2, 24 in the OV prosody, 23 in the no prosody condition. They received 100% exposure to English according to parental report. Parents gave informed consent before participation. The study was approved by the Behavioural Research Ethics Board of the University of British Columbia. Material An artificial grammar with an ambiguous underlying structure was created for Experiments 1 and 2. A four-syllable-long basic unit AXBY was concatenated repeatedly. The A and B categories had one token each, while the X and Y categories contained 9 tokens, making individual X and Y tokens 9 times less frequent than the A and B tokens. The lexicon of the artificial grammar consisted of the following words: A: fi , B: ge ; X: ru , pe , du , ba , fo , de , pa , ra , to , Y: mu , ri , ku , bo , bi , do , ka , na , ro (see also Fig. 3 ). This basic structure gave rise to a continuous stream of strictly alternating frequent (A and B) and infrequent (X and Y) words, mimicking function words and content words, respectively. The initial and final 15 s of the stream were ramped in amplitude in order to mask any phase information. The familiarization stream was thus ambiguous between a frequent word initial or FI (for example, AXBY) and a frequent word final or IF (for example, XBYA) parse. The familiarization stream was synthesized using the fr4 female diphone database of MBROLA [31] . In the OV prosody condition of Experiments 1 and 2, we used high pitch (224 Hz) on the prominent infrequent words and low pitch (200 Hz) on the non-prominent frequent words, both with a constant phoneme duration of 120 ms. In the VO prosody condition of Experiment 1, the prominent infrequent words were long (144 ms), the non-prominent frequent words were short (120 ms), and both had a constant pitch of 200 Hz. In the no prosody condition of Experiment 2, pitch and phoneme duration were held constant at 200 Hz and 120 ms, respectively. The test items were eight four-syllabic chunks from the stream ( Fig. 3 ). Four of them instantiated the FI order, the other four the IF order. Procedure In the head turn preference procedure [32] , the infant was seated on a caregiver’s lap in a sound-attenuated, dimly lit cubicle with one central and two side panels (see also Fig. 4 ). A light was mounted on each panel and loudspeakers were placed behind the side panels. A camera behind the central panel recorded the infant’s looking behaviour through a small hole under the central light. The tape was used for subsequent off-line coding of the infant’s looking behaviour. The caregiver wore dark glasses and listened to masking music over headphones to avoid any parental influence on the infant’s behaviour. During the experiment, an experimenter, blind to the stimuli and seated outside the testing cubicle, monitored infants’ looking behaviour and controlled the lights and the stimuli. During familiarization, the artificial grammar speech stream was played continuously from both loudspeakers. The lights blinked contingently upon the infant’s looking behaviour, but had no correlation with the speech stream. In the test, each trial began with the central light blinking to attract the infant’s attention. Once the infant fixated centrally, this light was extinguished and one of the side lights was turned on. When the infant stably fixated on the blinking side light (defined as a 30° head turn towards the side), the associated test item started playing from the loudspeaker on the corresponding side. The sound file continued until the end (22 s) or until the infant looked away for more than 2 s. After this, a new trial began. In total, the test phase consisted of eight test trials. How to cite this article: Gervain, J and Werker, J.F. Prosody cues word order in 7-month-old bilingual infants. Nat. Commun. 4:1490 doi: 10.1038/ncomms2430 (2013).